Kinetic modulation of a disordered protein domain by phosphorylation Phosphorylation is a major post-translational mechanism of regulation that frequently targets disordered protein domains, but it remains unclear how phosphorylation modulates disordered states of proteins. Here we determine the kinetics and energetics of a disordered protein domain the kinase-inducible domain (KID) of the transcription factor CREB and that of its phosphorylated form pKID, using high-throughput molecular dynamic simulations. We identify the presence of a metastable, partially ordered state with a 60-fold slowdown in conformational kinetics that arises due to phosphorylation, kinetically stabilizing residues known to participate in an early binding intermediate. We show that this effect is only partially reconstituted by mutation to glutamate, indicating that the phosphate is uniquely required for the long-lived state to arise. This mechanism of kinetic modulation could be important for regulation beyond conformational equilibrium shifts. Post-translational modifications in proteins participate in many fundamental cellular processes [1] , [2] , [3] and affect at least one-third of all eukaryotic proteins [4] , [5] . In particular, protein phosphorylation plays key roles in many signal-transduction processes [4] , [5] , [6] , [7] , [8] , preferentially targeting intrinsically disordered protein domains (IDPs) [4] , [5] . IDPs remain largely unstructured under native conditions [9] , resembling random-coil polymers akin to the unfolded states of proteins. Being present in >50% of eukaryotic proteins [10] , [11] , IDPs perform a plethora of biological functions [12] , [13] , [14] and are commonly associated with a variety of human diseases [15] , [16] , [17] , [18] . The effect of phosphorylation in proteins is manifold. For example, it can induce conformational changes [19] , promote order–disorder transitions [20] and modulate binding via electrostatic interactions with partners [21] . However, it remains largely unexplored whether phosphorylation can regulate the conformational kinetics of proteins, and what effect this may have on molecular recognition with other partners. This is especially interesting for protein domains that do not have a native folded conformation, and also difficult to address as it requires the characterization of low populated, transient states. In an attempt to understand how phosphorylation modulates disordered states of proteins, we determined the conformational kinetics and energetics of a disordered protein domain before and after phosphorylation at atomic resolution. We chose to study an experimentally well-characterized disordered fragment of the kinase-inducible domain (KID) of transcription factor CREB [22] (residues 116–147). KID includes the binding motif to the KIX domain of the coactivator CBP [23] ( Fig. 1b ). KID is known to be disordered in solution and form two alpha helices on binding [23] , a process that involves binding intermediates [24] . Molecular recognition of KID is regulated via phosphorylation of serine 133 in the αB helix, which increases its binding affinity 40-fold [25] (binding of residues 119–147 to KIX). Interestingly, phosphorylation barely affects the fraction of folded αA and αB helices [26] . Regulation of binding affinity is mostly ascribed to phosphate electrostatic and hydrogen bonding interactions with KIX. However, mutation of serine 133 to a negatively charged residue such as glutamate (often considered to mimic interactions with amide NH, lysine and arginine residues [27] ) cannot recapitulate pKID activity [28] . 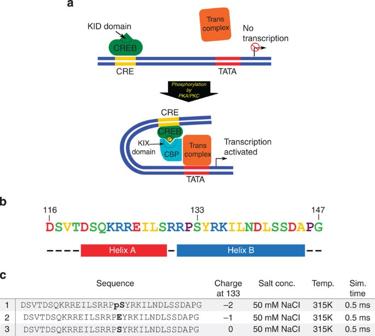Figure 1: System Overview. (a) Schematic representation of CREB activation. On phosphorylation of CREB at serine 133 at the kinase-inducible domain (KID), the KIX domain of the coactivator CBP binds to pKID with 40-fold increased affinity25and promotes transcriptional activation by recruiting the transcription machinery. (b) KID sequence with residues colour coded as positive (blue) and negatively (red) charged, polar (green) and hydrophobic (yellow). Helical regions formed in the complex with KIX23are shown. (c) Summary of simulations performed in this work. Figure 1: System Overview. ( a ) Schematic representation of CREB activation. On phosphorylation of CREB at serine 133 at the kinase-inducible domain (KID), the KIX domain of the coactivator CBP binds to pKID with 40-fold increased affinity [25] and promotes transcriptional activation by recruiting the transcription machinery. ( b ) KID sequence with residues colour coded as positive (blue) and negatively (red) charged, polar (green) and hydrophobic (yellow). Helical regions formed in the complex with KIX [23] are shown. ( c ) Summary of simulations performed in this work. Full size image All-atom, explicit solvent micro to millisecond MD simulations [29] , [30] , [31] have in recent years significantly contributed to our understanding of disordered states of proteins [29] , [30] , [32] , [33] . Computational studies on KID protein using replica exchanged implicit solvent MD simulations [34] , and short all-atom MD simulations [35] showed that KID is largely unstructured and phosphorylation barely affects its helical propensity. Moreover, coarse grain and short, high-temperature all-atom simulations suggested that binding of KID to KIX initiates at the αB helix [35] , [36] , [37] , [38] . However, difficulties in resolving the micro to millisecond timescale using all-atom, unbiased MD simulations impeded the assessment of the effect of phosphorylation on long-time scales and thus on conformational kinetics. Here, we use all-atom, explicit solvent molecular dynamic (MD) simulations and resolve equilibrium by performing 1.7 ms of aggregated simulation time on the distributed computing network GPUGRID.net [39] with ACEMD [40] . We identify a metastable, partially ordered state with a 60-fold slowdown in conformational kinetics, exchanging at the multi-microsecond time regime, present only in phosphorylated KID. This post-translational modification kinetically locks residues in helix αB that participates in an early binding intermediate, while no significant change in the population of the ordered state was observed. Our results are in line with previous experimental NMR analyses. We suggest that long-lived states favoured by phosphorylation are partially responsible for the increased binding affinity of pKID to KIX and propose that kinetic modulation of disordered protein domains may be an important mechanism of regulation by phosphorylation at the biochemical level beyond conformational equilibrium shifts. Induction of slow conformational exchange by phosphorylation To study the effect of phosphorylation on the KID domain of CREB we performed all-atom, explicit solvent MD simulations with 1.7 ms of total aggregated data for the following systems: phosphorylated KID at serine 133 (pKID), KID domain and a S133E mutant (gKID) used as a control ( Fig. 1 ; see Methods). For each system, the data were analysed by constructing a Markov state model (MSM) of the entire ensemble of trajectories (see Methods). MSMs have been used previously to successfully calculate several slow processes from ensemble MD simulations [41] , [42] , [43] , [44] , [45] . We used inter-residue Cα-Cα distances and φ/ψ backbone dihedral angles as general metrics to build the kinetic model. The conformational space was discretized into 1,000 clusters and then projected on a 5-dimensional space using a new dimensionality reduction technique (time-sensitive independent component analysis [46] ), which identifies the slow coordinates in the dynamics. The characteristic relaxation timescales of the first and second slowest processes for pKID, KID and gKID proteins, as determined from the Markov model, are reported in Table 1 . The slowest relaxation process of pKID and KID differs by 60-fold (37 versus 0.6 μs). The second slowest process of pKID is also an order of magnitude slower than the slowest process observed in KID. To assess whether that slowdown in conformational kinetics was specific of the phosphate, we mutated the serine 133 to glutamate to partially mimic the negatively charged phosphate group [27] . The slowest process in gKID was found well below that of pKID ( Table 1 ). Therefore, phosphorylation induced a slow exchange process in the multi-microseconds time regime, a kinetic fingerprint of pKID that could not be recapitulated by S133E mutation. Table 1 Timescales of 1st and 2nd slowest processes for the systems studied. Full size table Identification of a metastable state in phosphorylated KID As the slowest process for all systems is well separated from the rest, we used a simple, two-state kinetic model to analyse conformational transitions in KID, called D (disordered) and O (ordered), where τ 1 and τ −1 are the forward and backward mean first passage times. The relaxation time ( τ ex ) is defined as τ ex =( τ 1 −1 + τ −1 −1 ) −1 . We obtained a kinetic clustering over just two states using the Perron-cluster cluster analysis [47] . The slowest exchange process identified in pKID, that occurs at 37±1 μs ( Table 1 ), had a forward ( τ 1 ) and backward ( τ −1 ) transition time of 463±22 and 37.0±0.8 μs ( Fig. 2 , Supplementary Fig. 1 ). The stationary (equilibrium) populations obtained from the Markov model are 95±1 and 5±1%. Statistical errors were determined using a bootstrapping procedure of the data (see methods). 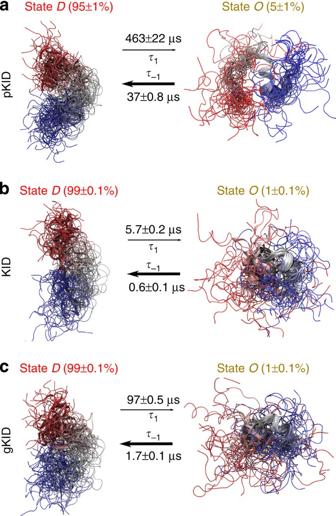Figure 2: Kinetic modulation of the energy landscape in a disordered domain via phosphorylation. Conformational exchange between stateD(disordered) and stateO(ordered) is shown together with forward (τ1) and backward (τ−1) transition times for (a) pKID, (b) KID and (c) gKID (see alsoSupplementary Fig. 1). Conformations were aligned using residues with the lowest Cα-Cα distance variance. Error estimates were determined using a bootstrapping technique (see Methods). N- to C terminal is colour coded red and blue. Figure 2: Kinetic modulation of the energy landscape in a disordered domain via phosphorylation. Conformational exchange between state D (disordered) and state O (ordered) is shown together with forward ( τ 1 ) and backward ( τ −1 ) transition times for ( a ) pKID, ( b ) KID and ( c ) gKID (see also Supplementary Fig. 1 ). Conformations were aligned using residues with the lowest Cα-Cα distance variance. Error estimates were determined using a bootstrapping technique (see Methods). N- to C terminal is colour coded red and blue. Full size image For the case of non-phosphorylated KID, we found a large state that accounted for most of the population (99±0.1%, Fig. 2 ). The slowest transitions in KID occurred at 0.6±0.01 μs ( Table 1 ), with forward and backward transition times of 5.7±0.2 and 0.6±0.1 μs ( Fig. 2 , Supplementary Fig. 1 ). Control simulations with gKID (S133E) protein also showed a largely populated state (99±0.1%) and a slow exchange process of 1.8±0.01 μs ( Supplementary Fig. 1 ). Phosphorylation of KID resulted in a 60-fold slowdown exchange process ( τ ex ~37 μs) as compared with KID domain ( τ ex ~0.6 μs) and affected the forward (state D to state O ) and backward (state O to state D ) transition times by a factor of 80 and 60, respectively. Phosphorylation kinetically locks binding residues To further investigate the slowdown observed on conformational exchange in pKID as compared with both KID and gKID proteins, we computed the autocorrelation function (ACF) for helix folding and unfolding at the residue level and determined the characteristic relaxation times ( Fig. 3a , see Methods, Supplementary Fig. 3 ). We found that residues 131–136 at the N-terminal part of αB helix undergo slow multi-microsecond conformational exchange ( τ ex ~40 μs) and, therefore, participate in the slowest process observed in pKID ( Table 1 ). NMR experiments identified an early intermediate complex in which N-terminal αB region is engaged with KIX [24] . This region maps on top of residues undergoing slow exchange in phosphorylated KID ( Fig. 3a ). It is plausible, therefore, that the state O identified in this work and the early binding intermediate detected by NMR have common structural details. 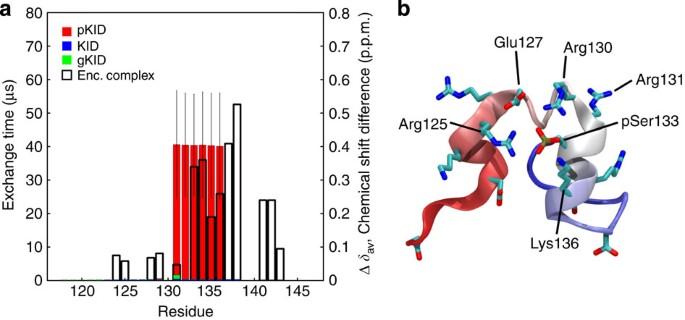Figure 3: Identification of residues undergoing slow conformational exchange in phosphorylated KID. (a) Residue-specific relaxation times of helix folding/unfolding process (filled bars) derived from autocorrelation functions. Empty bars show CS changes in pKID that map residues participating in an early binding intermediate as detected by NMR24. Error bars represent the s.e.m. as determined by bootstrapping (see Methods). (b) Example of a kinetically locked conformation in phosphorylated KID. The peptide backbone is shown in cartoon representation. Heavy atoms of phosphorylated serine 133 and several charged residues are shown as sticks. Figure 3: Identification of residues undergoing slow conformational exchange in phosphorylated KID. ( a ) Residue-specific relaxation times of helix folding/unfolding process (filled bars) derived from autocorrelation functions. Empty bars show CS changes in pKID that map residues participating in an early binding intermediate as detected by NMR [24] . Error bars represent the s.e.m. as determined by bootstrapping (see Methods). ( b ) Example of a kinetically locked conformation in phosphorylated KID. The peptide backbone is shown in cartoon representation. Heavy atoms of phosphorylated serine 133 and several charged residues are shown as sticks. Full size image Structural analysis As expected for an IDP, the most populated state in pKID, KID and gKID is largely unstructured ( Supplementary Fig. 2 ). We observed an increase in the population of the minor state from 1±0.1 to 5±1% when serine 133 was phosphorylated and no change on S133E mutation ( Fig. 2 ). In all cases the state was characterized by an increase in helical content of residues in αB helix ( Supplementary Fig. 2 ). This minor state is referred herein as ordered or state O . This effect was most notable for the case of pKID, in which ~80% of the conformers in this state had the N-terminal residues 131–135 of αB helix folded. An interesting structural feature of states O and D is that they group conformations in which residue 131 is either forming part of the αB helix or unfolded, respectively. This structural signature separates states that exchange slowest in all three systems. Interestingly, NMR relaxation experiments showed that residue 131 in pKID folds one to two orders of magnitude slower than the rest of residues in the complex with KIX [24] . The helicity of residues in αB helix tends to increase in this state with respect to the disordered state D ( Supplementary Fig. 2 ). Overall, the slow exchange processes involved disordered (state D )–ordered (state O ) transitions. Inspection of state O in pKID revealed additional features beyond secondary structure formation ( Fig. 3b ). The phosphate moiety, located within residues undergoing slow exchange, serves as a staple that locks pKID into a conformation with the αA helix partially folded (~35%) and the N terminal of αB helix mostly folded (~80%) ( Supplementary Fig. 2 ). In addition, a turn bridging helix αA and αB is held by electrostatic interactions and hydrogen bonds between the phosphate in helix αB and lysine and arginine residues in the C-terminal region of αA helix. Note that similar states are also observed for KID and gKID proteins, but these states exchange fast with the rest of the conformations. Other types of secondary structural arrangements were also present, such as beta sheets, but these were low populated (<0.1%) and exchanged rapidly with other states (faster than 500 ns for the case of pKID, for example). Comparison with NMR We assessed the structural properties of our equilibrium simulations by a direct comparison with backbone chemical shifts (CS) measured by NMR spectroscopy for KID and pKID proteins [26] . CS allows mapping secondary structure propensities in disordered states of proteins. Overall, results were found in agreement with experimental CS ( Fig. 4 , Cα/Cβ RMSD NMR-MD for pKID and KID is 0.6/0.4 and 0.5/0.4 p.p.m., error in the prediction algorithm is ~0.5 p.p.m. for SHIFTX2 (ref. 48 ) and ~1 p.p.m. for SPARTA+ (ref. 49 )). A deviation between calculated and measured Cα CS was observed for residues 120–128 ( Fig. 4a ), indicating an increased population of helix αA present under experimental conditions (288 versus 315 K used for simulations). However, there is a known α-helical induction of structure in KID at low temperatures [50] , so the difference might be due to this or limitations of the force fields. We note that CS could not be calculated for pSer133, which was then mutated to serine, affecting prediction of neighbouring residues 132 and 134. Comparison of CS changes induced by phosphorylation ( Fig. 4b ) showed a similar pattern between calculated and measured CS. These findings suggested common structural rearrangements of KID on phosphorylation as determined by simulation and NMR. 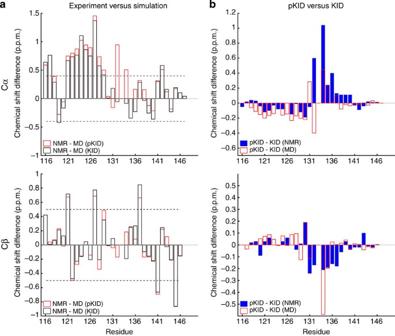Figure 4: Comparison against NMR data. (a) Chemical shift (CS) difference between experimentally measured (NMR, 288 K) and calculated (MD, 315 K). Calculations were performed with SPARTA+ (ref.49) and SHIFTX2 (ref.48), which rendered equivalent results. Dashed lines correspond to the intrinsic error in the prediction estimated from SHIFTX2 (Cα and Cβ errors are 0.4 and 0.5 p.p.m., for SPARTA+ the estimated errors are ~1 p.p.m.). Cα/Cβ RMSD for pKID and KID is 0.6/0.4 and 0.5/0.4 p.p.m. (b) Experimental (NMR, blue) and calculated (MD, red) CS differences between pKID and KID systems. Note that calculations in pKID were performed with serine 133 instead of phosphorylated serine 133, affecting prediction of neighbouring residues 132 and 134. Figure 4: Comparison against NMR data. ( a ) Chemical shift (CS) difference between experimentally measured (NMR, 288 K) and calculated (MD, 315 K). Calculations were performed with SPARTA+ (ref. 49 ) and SHIFTX2 (ref. 48 ), which rendered equivalent results. Dashed lines correspond to the intrinsic error in the prediction estimated from SHIFTX2 (Cα and Cβ errors are 0.4 and 0.5 p.p.m., for SPARTA+ the estimated errors are ~1 p.p.m.). Cα/Cβ RMSD for pKID and KID is 0.6/0.4 and 0.5/0.4 p.p.m. ( b ) Experimental (NMR, blue) and calculated (MD, red) CS differences between pKID and KID systems. Note that calculations in pKID were performed with serine 133 instead of phosphorylated serine 133, affecting prediction of neighbouring residues 132 and 134. Full size image Experimental NMR measurements detected similar inter-proton NOE distance patterns for the phosphorylated and non-phosphorylated forms of the domain except in the vicinity of the phosphorylation site. Six weak or very weak NOEs that involved residues 127, 131, 134 and 137 were only observed for pKID [26] . Overall, NOE distances are similar for KID and pKID (4.8±0.6 Å). NOEs involving I127H N -R130H N and I131H N -R133H N nuclei showed smaller distances for KID (Δ dist =0.3±0.1 Å). NOE distances involving residues R131Hα-Y134H N and Y134Hα-I137H N were by contrast smaller for the case of pKID (Δ dist =0.5±0.1 Å). These additional NOEs bridged up to seven residues. This NOE pattern suggested an increase in helical content near the N-terminus of the αB helix, in agreement with NMR. We have described the conformational kinetics and energetics of an intrinsically disordered protein domain, the KID domain of the transcription factor CREB, before and after a post-translational phosphorylation. We identified the presence of a metastable, partially ordered state with at least 60-fold slowdown in conformational exchange that arises due to phosphorylation, involving folding and unfolding of residues in the N-terminal region of αB helix. Previous NMR studies investigating conformational dynamics of KID in its unbound state [24] can detect exchange processes in the ~0.3–10 ms time window [51] and, therefore, the process we observe in this work (tens of microseconds) remained hidden. Phosphorylation induced a minor shift (in absolute terms) in the equilibrium distribution of folded αA and αB helices, in agreement with NMR data [24] . However, an 80- and 60-fold increase in the folded and unfolded residence time for residues at the N-terminal αB helix was observed. These N-terminal αB residues were found by NMR experiments to participate in an early binding intermediate [24] . Binding of kinetically locked regions can give other transient interactions time to form, potentially increasing the number of productive binding events and thus the overall affinity for the binding partner. Similarly, kinetically locked regions that participate in molecular recognition could frustrate the unbinding process. This would result in a shift of the binding equilibrium towards the bound state. We devised a toy kinetic model to show that, at least in principle, a slowdown in conformational kinetics of both forward and backward transition rates by the same amount can translate into a 40-fold increase in binding affinity ( Fig. 5 ). In an analogy to the binding mechanism of KID ( D ) to KIX ( X ), in our model the bound complex ( XD ) is formed via an intermediate [24] . A key element of the model is the presence of productive ( XD p ) and nonproductive ( XD np ) intermediates, for which phosphorylation induces a 100-fold slowdown in conformational exchange. It is therefore reasonable to propose that the slowdown in conformational exchange we observed offers an additional mechanism to increase binding affinity. The fact that the glutamate mutation cannot sustain long-lived states and disrupts [25] the binding is consistent with this proposed mechanism of modulation. 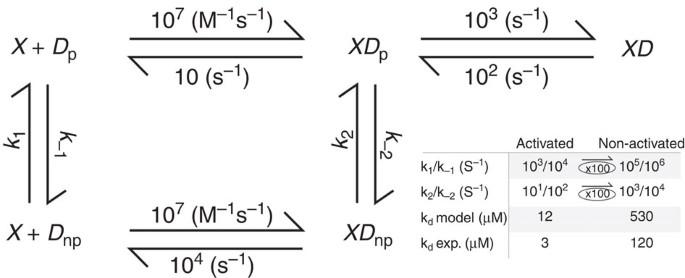Figure 5: Illustrative example on the potential role of conformational kinetics in overall binding affinity. In this example unbound species exchange between two states, labelledDpandDnp. Phosphorylation induces a 100-fold slowdown in conformational kinetics, affecting forward (k1) and backward (k−1) rates by the same amount. A key element of the model is binding via productive (XDp) and non-productive (XDnp) intermediates, for which phosphorylation induces a 100-fold conformational exchange slowdown (k2andk−2). Unbinding of non-productive (XDnp) intermediate is faster than unbinding ofXDp(1,000-fold, a leakage route). Exchange for productive and nonproductive intermediates is set 100 times slower than that in their free state. This example results in 40-fold increased binding affinity for activated (for example, phosphorylated) protein. Figure 5: Illustrative example on the potential role of conformational kinetics in overall binding affinity. In this example unbound species exchange between two states, labelled D p and D np . Phosphorylation induces a 100-fold slowdown in conformational kinetics, affecting forward ( k 1 ) and backward ( k −1 ) rates by the same amount. A key element of the model is binding via productive ( XD p ) and non-productive ( XD np ) intermediates, for which phosphorylation induces a 100-fold conformational exchange slowdown ( k 2 and k −2 ). Unbinding of non-productive ( XD np ) intermediate is faster than unbinding of XD p (1,000-fold, a leakage route). Exchange for productive and nonproductive intermediates is set 100 times slower than that in their free state. This example results in 40-fold increased binding affinity for activated (for example, phosphorylated) protein. Full size image Previous studies have shown that pSer133 contributes to binding via specific intermolecular contacts, and a loss of affinity is seen when mutating specific residues in KIX [25] , [28] , [52] . The exact atomistic mechanism and whether these contacts are also sufficient alone for binding is less clear. In our kinetic model, multiple routes are possible. A mutation destabilizing some important contacts would reduce the residence time of the bound form (1/ k −5 in the kinetic diagram). The effect can be easily simulated, and a 10 times increase in k −5 corresponds to 10 times lower affinity. However, the additional kinetic route is also mathematically viable, that is, the binding affinity can be modulated controlling the time spent in productive versus non-productive intermediates. Both routes can play a role in general, and usually there is a complementary effect in such complex processes. The fact that it is generally possible to modulate binding of a disordered domain in a kinetic way is novel and practical. In our case, it was indeed suggested by the fact that we see a slowdown in conformational kinetics of pKID, which is not seen in gKID. It has also been proposed that pSer133 could reduce the conformational entropy of the unbound state of KID [34] , [53] . This is compatible with the results presented here. Phosphorylation of KID could change conformational entropy due to altered kinetics, but compensate in conformational enthalpy producing similar overall populations. With disordered domains taking part in >50% of proteins responsible for signalling in the cell [54] , this kinetic mechanism of modulation highlights a further possible mechanism by which post-translation modifications may affect disordered domains and their interactions with binding partners. Simulation setup The sequence corresponding to residues 116–147 of CREB was used in this work ( Fig. 1 ). Initial coordinates were built using VMD software [55] . CHARMM22* (ref. 56 ) force field was used for the peptides. The phosphate group on pKID (bearing two negative charges) was patched using that provided in the CHARMM27 (ref. 57 ) force field with serine parameters from CHARMM22*. TIP3P model was used for the water molecules. The peptides were placed in a cubic water box of 64-angstrom sides and equilibrated for 2 ns at 315 K in the NPT ensemble at 1 bar. The peptides were simulated at 500 K for 120 ns to decorrelate from the initial conformation at constant volume (no cis conformations of peptide bonds were observed). For each of the three simulated systems, 100 starting structures were taken from each nanosecond of the last 100 ns of the high-temperature run. For each of those 100 starting structures, 10 replicas were submitted to GPUGRID.net [39] using ACEMD [40] . An additional 200 simulations were later performed for each system to ensure adequate sampling of the process described, for a total of 1,200 for each system. Production runs lasted 480 ns and were performed at 315 K in the NVT ensemble. For all simulations, the particle mesh Ewald algorithm [58] , rigid hydrogen bonds, hydrogen mass repartitioning [59] and a time step of 4 fs were employed. MSM analysis We built a MSM from the molecular simulation trajectories. MSMs have been successfully used to reconstruct the equilibrium and kinetic properties in a large number of molecular systems [41] , [44] , [60] , [61] , [62] . By determining the frequency of transitions between conformational states, we construct a master equation that describes the dynamics between a set of conformational states. Relevant states are determined geometrically by clustering the simulation data onto a metric space (for example, contact maps). The projected space used in this work is formed by the distances between all 32 Cα pairs plus φ/ψ backbone dihedral angles of the KID peptide. This high-dimensional data were then projected into five dimensions using the time-sensitive independent component analysis method [46] with a 2-ns lag time, which selects the slowest varying variables. The data were then clustered into 1,000 states using the k-means clustering algorithm. Results remained consistent with changes in the number of clusters (for example, 10 4 ) and on the projected dimensions (for example, 10 dimensions). The master equation is then built as where P i ( t ) is the probability of state i at time t , and k ij are the transition rates from j to i , and K =( K ij ) is the rate matrix with elements K ij = k ij for i ≠ j and K ii =−∑ j ≠ i k i . The master equation d P /d t = KP has solution with initial condition P (0) given by P ( t )= T ( t ) P (0), where we defined the transition probability matrix T ij ( t )=(exp[ K t ]) ij = p ( i , t | j ,0), that is, the probability of being in state i at time t , given that the system was in state j at time 0. In practical terms, p ij (Δ t ) is estimated from the simulation trajectories for a given lag time Δ t using a maximum likelihood estimator compatible with detailed balance [63] . The eigenvector π with eigenvalue 1 of the matrix T (Δ t ) corresponds to the stationary, equilibrium probability. Higher eigenvectors correspond to exponentially decaying relaxation modes [62] for which the relaxation timescale is computed by the eigenvalue as , where λ s is the largest eigenvalue above 1. For long enough lag times Δ t the model will be Markovian; however, every process faster than Δ t is lost. Therefore, the shortest lag is chosen for which the relaxation timescales do not show a dependence on the lag time Δ t anymore (See Supplementary Fig. 1 ). In our case, we chose a 100-ns lag time as it showed the least dependence for the slowest processes in all systems. Furthermore, the initial N microstates can be lumped together into macrostates using kinetic information from the MSM eigenvector structure [47] . This allows one to obtain a limited number of important, kinetically distinct states. Mean first passage times and commitor probabilities can also be calculated to obtain the relevant kinetics of the system [64] . Autocorrelation analysis A MSM-based trajectory of 10 ms effective time (100 ns lag time) was built for each system by sampling conformations according to transition probabilities between microstates (MSM trajectories are distributed on request to the authors). Relaxation times were calculated by fitting exponentials to ACFs. The fitting procedure included three exponentials. We used a time constant <100 ns for the first, which is the lag time used to build the kinetic model, to account for the initial fast decay in the ACF. The fitting was limited to the first 100 μs of the ACF. See Supplementary Methods for details. Error estimation We estimated errors for all properties using a bootstrapping technique. We performed 10 independent runs in which 20% of the trajectories were randomly eliminated and a new MSM was built before properties were recalculated. NMR calculations We calculated expected CS from the simulation using 10,000 frames of the MSM trajectory for each of the three simulations. Calculations with SHIFTX2 (ref. 48 ) and SPARTA+ (ref. 49 ) provided consistent results. Average NOE distances ( r ) were calculated from the MSM trajectories as < r −6 > −1/6 . Kinetic model We built a kinetic model based on five coupled reactions ( Fig. 5 and Supplementary Methods ). As with a previously described mechanism for KID binding to KIX [24] , we used an intermediate step. Unlike previous models, our model contains an additional state for both the unbound and intermediate states, such that a binding competent and incompetent conformer (termed productive and non-productive, respectively) can be accounted for. We label the exchange between these states reaction 1 (rate k ±1 ) in the unbound state and reaction 2 in the intermediate state (rate k ±2 ). Kinetic rates for the other step reactions 3, 4 and 5 (rates k ±3 , k ±4 , k ±5 ) were taken from those determined by NMR. The coupled equations were solved numerically using MATLAB. The equilibrium dissociation constant was calculated as K d =[ D free ][ X free ]/[ XD ]. How to cite this article: Nathaniel, S. et al . Kinetic modulation of a disordered protein domain by phosphorylation. Nat. Commun. 5:5272 doi: 10.1038/ncomms6272 (2014).